MacroH2A histone variants act as a barrier upon reprogramming towards pluripotency The chromatin template imposes an epigenetic barrier during the process of somatic cell reprogramming. Using fibroblasts derived from macroH2A double knockout (dKO) mice, here we show that these histone variants act cooperatively as a barrier to induced pluripotency. Through manipulation of macroH2A isoforms, we further demonstrate that macroH2A2 is the predominant barrier to reprogramming. Genomic analyses reveal that macroH2A1 and macroH2A2, together with H3K27me3, co-occupy pluripotency genes in wild-type (wt) fibroblasts. In particular, we find macroH2A isoforms to be highly enriched at target genes of the K27me3 demethylase, Utx, which are reactivated early in iPS reprogramming. Finally, while macroH2A dKO-induced pluripotent cells are able to differentiate properly in vitro and in vivo , such differentiated cells retain the ability to return to a stem-like state. Therefore, we propose that macroH2A isoforms provide a redundant silencing layer or terminal differentiation ‘lock’ at critical pluripotency genes that presents as an epigenetic barrier when differentiated cells are challenged to reprogram. MacroH2A isoforms are unique H2A histone variants due to the presence of a 30-kDa non-histone domain (macro domain) at their C-termini [1] . MacroH2A variants are generally considered transcriptionally repressive in nature due to their association with forms of condensed chromatin such as the inactive X chromosome (Xi) [2] , [3] , [4] , [5] , [6] , and inactive genes [7] , [8] , [9] , [10] . MacroH2A1 and macroH2A2 isoforms are encoded by two distinct genes (H2AFY and H2AFY2, respectively), and macroH2A1 is alternatively spliced, resulting in two macroH2A1 isoforms, macroH2A1.1 and macroH2A1.2, that differ by only one exon in the macro domain [11] . The pluripotent stem cell state is under the control of a highly regulated transcriptional circuitry [12] , that is complemented by chromatin regulation [13] . Embryonic stem cell (ESC) chromatin is considered to be more ‘open’ than that of its differentiated progeny, with robust chromatin remodelling activities to allow for efficient chromatin reorganization that occurs during lineage specification [14] , [15] , [16] . In keeping with this, deposition of macroH2A1 is globally enriched in differentiated cells as compared with their pluripotent counterparts [17] . Two recent studies have probed macroH2A isoforms in the context of ESC pluripotency via RNA interference. Both demonstrated that macroH2A isoforms are dispensable for self-renewal, however they conflicted on the role of macroH2A during differentiation. While one study showed that loss of macroH2A isoforms inhibits proper differentiation [18] , another reported that macroH2A-deficient ESCs executed X inactivation efficiently and were able to effectively differentiate towards multiple lineages [19] . Thus, the role of macroH2A in ESC differentiation remains ambiguous, as it has yet to be examined in the context of genetically deficient mice [8] , [20] . MacroH2A isoforms have also been studied in the context of reprogramming via somatic cell nuclear transfer (SCNT). Intriguingly, macroH2A is rapidly removed from the mammalian somatic cell nucleus upon transplantation into mouse oocytes [21] , [22] , [23] . Using an alternative system of SCNT, Gurdon and colleagues [24] implicated macroH2A as a factor conferring resistance to Xi reactivation of differentiated mammalian nuclei when transferred into Xenopus oocytes. Pluripotent cells can also be generated via ectopic expression of key pluripotency-related transcription factors (TFs) in somatic cells in order to generate induced pluripotent stem cells (iPSCs) [25] . However, the epigenome imparts a barrier during the reprogramming process towards pluripotency [26] , [27] . We previously hypothesized that histone variants may act as an epigenetic barrier during somatic cell reprogramming because they are generally incorporated into chromatin in a replication-independent manner, and thus may mark particular genomic regions in fully differentiated cells [27] . Here, we have examined the contribution of macroH2A isoforms via induced pluripotency using genetically engineered mouse models deficient for both macroH2A1 and macroH2A2. We find that while macroH2A isoforms act cooperatively, macroH2A2 acts as the predominant epigenetic barrier when somatic cells are challenged to reprogram. During normal ESC differentiation and in development, macroH2A isoforms are globally incorporated into chromatin, and deposited at pluripotency genes, such as the Oct4 locus, a master regulator of pluripotency [28] . While we demonstrate that macroH2A isoforms are not required for inactivating the pluripotency genes (due to redundant silencing mechanisms), we find that macroH2A and its highly associated histone modification, H3K27me3, are enriched at a set of Utx target genes required for the early stages of induced pluripotency. We suggest that the presence of macroH2A at these genes acts to prevent reactivation of critical pluripotency genes in differentiated cells, thus creating a barrier to reprogramming. macroH2A is dynamic during differentiation and reprogramming We investigated the levels of both macroH2A1 and macroH2A2 isoforms in the histone and chromatin fractions of ESCs induced to differentiate by multiple methods. We observed increased macroH2A1 and macroH2A2 in the histone fraction of ESCs differentiated by retinoic acid (RA) ( Fig. 1a ), which was corroborated by quantitative mass spectrometry (qMS) [29] ( Fig. 1b ). Using embryoid body (EB) formation assays, we detected similar global histone changes in the chromatin fraction ( Fig. 1c ). We also observed similar results by comparing ESCs with distinct differentiated cell types such as mouse embryonic fibroblasts (MEFs) and dermal fibroblasts (DFs) ( Fig. 1d ). Collectively, these data suggest that macroH2A isoforms are specifically deposited into chromatin upon differentiation, as well as during mouse development. Of note, we also observed a decrease in H2A.Z levels in these studies, suggesting that macroH2A and H2A.Z histone variants might have distinct roles during ESC differentiation. 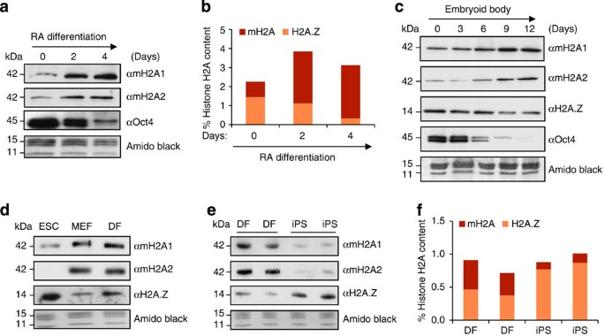Figure 1: macroH2A chromatin deposition increases upon differentiation and is lost upon reprogramming. (a) Acid extracted histones from RA-differentiated CCE ESCs probed for macroH2A isoforms. Chromatin-bound Oct4 is used to confirm differentiation; Amido black of core histones used for loading. (b) Histone H2A variant composition as analysed by qMS during ESC RA-induced differentiation. Values represented as percentage of total H2A; two biological replicates, six technical replicates shown. (c) Chromatin fraction of EB time course (E14 ESCs) used to probe H2A variants. Oct4 is used to confirm differentiation; Amido black of core histones used for loading. (d) Chromatin fraction of CCE ESC, MEFs and DFs probed for H2A variants. (e) Wt mouse DFs and their iPS-reprogrammed counterparts probed for H2A variants. (f) qMS analysis of macroH2A and H2A.Z using histones isolated from cells used ine. Figure 1: macroH2A chromatin deposition increases upon differentiation and is lost upon reprogramming. ( a ) Acid extracted histones from RA-differentiated CCE ESCs probed for macroH2A isoforms. Chromatin-bound Oct4 is used to confirm differentiation; Amido black of core histones used for loading. ( b ) Histone H2A variant composition as analysed by qMS during ESC RA-induced differentiation. Values represented as percentage of total H2A; two biological replicates, six technical replicates shown. ( c ) Chromatin fraction of EB time course (E14 ESCs) used to probe H2A variants. Oct4 is used to confirm differentiation; Amido black of core histones used for loading. ( d ) Chromatin fraction of CCE ESC, MEFs and DFs probed for H2A variants. ( e ) Wt mouse DFs and their iPS-reprogrammed counterparts probed for H2A variants. ( f ) qMS analysis of macroH2A and H2A.Z using histones isolated from cells used in e . Full size image Next we questioned whether macroH2A isoforms are removed from the chromatin fraction upon somatic cell reprogramming. Therefore, we used the Cre-excisable Stemcca polycistronic lentivirus encoding Oct4, Sox2, Klf4 and Myc (OSKM) [30] to reprogram multiple batches of DFs isolated from wt Sv/129 mice. We observed that macroH2A1 and macroH2A2 levels are lower in the chromatin fraction of iPSCs when compared with the DFs, while H2A.Z levels are increased ( Fig. 1e ), and qMS analysis confirmed our immunoblot results ( Fig. 1f ). Together, these results suggest that low levels of macroH2A contribute to the pluripotent state and that macroH2A isoforms might act as a barrier to iPS reprogramming in somatic cells. Characterization of macroH2A knockout DFs In order to address this hypothesis, we isolated DFs from both wt and macroH2A1- and macroH2A2-deficient newborn mice (dKO mice) ( Fig. 2a ; Supplementary Fig. S1a ). These dKO mice are viable and free of obvious developmental defects (J.R.P., manuscript in preparation). Both male and female DFs were isolated in order to account for any potential sex differences that might be revealed during iPS reprogramming, as macroH2A coats the Xi in differentiated female cells ( Fig. 2a ). 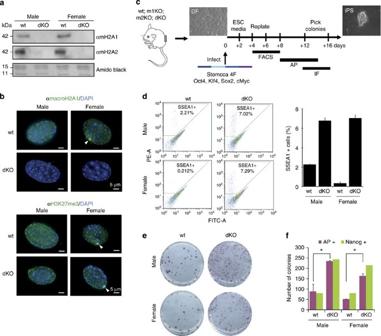Figure 2: macroH2A deficiency improves iPS reprogramming efficiency. (a) Chromatin extracts from wt and dKO DFs probed for macroH2A1 and macroH2A2; Amido black of core histones used for loading. (b) Immunofluorescence of macroH2A1 (top) and H3K27me3 (bottom) in wt and dKO male and female DFs. Note loss of macroH2A staining in dKO cells and enrichment of H3K27me3 at the Xi (white arrows) in female cells of both wt and dKO genotypes. DAPI used to stain DNA; Scale bar, 5 μm. (c) Experimental scheme of iPS reprogramming from DF (wt, m1KO, m2KO and dKO) to iPS colonies, using a polycistronic lentiviral vector (Stemcca) encoding four factors (4F): OSKM. Reprogramming efficiency was analysed by FACS analysis of SSEA1-positive cells, AP staining of iPS colonies, and IF for Nanog; time frame of experiments shown. (d) FACS plots for SSEA1-phycoerythrin-stained DFs showing increased percentage of SSEA1-positive cells in dKO (male and female) at 8 days post infection; quantitation on the right. (e) Representative wells of AP-positive iPS colonies, indicating increased reprogramming efficiency in dKO DFs at 14 days post infection. (f) Number of colonies (AP and Nanog positive) obtained at day 14 post infection; mean±s.d. (n=3); unpaired Student’s test (two tailed)P<0.05 (asterisk):P=0.05, male DFs (wt versus dKO);P=0.02, female DFs (wt versus dKO); Representative of six experiments with four biological replicates. Figure 2: macroH2A deficiency improves iPS reprogramming efficiency. ( a ) Chromatin extracts from wt and dKO DFs probed for macroH2A1 and macroH2A2; Amido black of core histones used for loading. ( b ) Immunofluorescence of macroH2A1 (top) and H3K27me3 (bottom) in wt and dKO male and female DFs. Note loss of macroH2A staining in dKO cells and enrichment of H3K27me3 at the Xi (white arrows) in female cells of both wt and dKO genotypes. DAPI used to stain DNA; Scale bar, 5 μm. ( c ) Experimental scheme of iPS reprogramming from DF (wt, m1KO, m2KO and dKO) to iPS colonies, using a polycistronic lentiviral vector (Stemcca) encoding four factors (4F): OSKM. Reprogramming efficiency was analysed by FACS analysis of SSEA1-positive cells, AP staining of iPS colonies, and IF for Nanog; time frame of experiments shown. ( d ) FACS plots for SSEA1-phycoerythrin-stained DFs showing increased percentage of SSEA1-positive cells in dKO (male and female) at 8 days post infection; quantitation on the right. ( e ) Representative wells of AP-positive iPS colonies, indicating increased reprogramming efficiency in dKO DFs at 14 days post infection. ( f ) Number of colonies (AP and Nanog positive) obtained at day 14 post infection; mean±s.d. ( n =3); unpaired Student’s test (two tailed) P <0.05 (asterisk): P =0.05, male DFs (wt versus dKO); P =0.02, female DFs (wt versus dKO); Representative of six experiments with four biological replicates. Full size image Next, we examined the staining pattern of macroH2A1 in the DFs. As expected, wt cells have macroH2A staining throughout the nucleus and an obvious Xi was observed in female cells. In contrast, no detectable nuclear staining was observed in the dKO cells of either sex ( Fig. 2b ). We also examined the staining pattern of H3K27me3, a facultative heterochromatic mark that tracks with macroH2A genomic binding and is enriched on the Xi [6] , [7] , [9] . Both female cells of wt and dKO origin retain an Xi as evidenced by H3K27me3 ( Fig. 2b ). These results are consistent with studies showing that loss of macroH2A1 does not reactivate the Xi [31] . As the efficiency of reprogramming can be affected by the proliferation rates of the starting somatic cells [32] , we examined the growth properties of wt and dKO DFs. Using proliferation assays, as well as 5-ethynyl-2'-deoxyuridine incorporation studies to detect cells in S phase, we did not find significant differences between wt and dKO DFs ( Supplementary Fig. S1b,c ). Thus, any potential differences observed upon reprogramming are not due to the initial proliferative state of the DFs. iPS reprogramming is enhanced in the absence of macroH2A Using these well-characterized DFs, we performed iPS studies using Stemcca polycistronic lentivirus encoding OSKM ( Fig. 2c ). By performing fluorescence-activated cell sorting (FACS) analysis for stage-specific embryonic antigen-1 (SSEA1), we observed a notable increase in the SSEA1+ population in macroH2A dKO cells early in the reprogramming process (4–8 days) ( Fig. 2d ). This suggests that loss of macroH2A isoforms facilitates the early stages of reprogramming. Alkaline phosphatase (AP) staining, which marks undifferentiated ES-like cells, demonstrated enhanced reprogramming in macroH2A dKO cells ( Fig. 2e ). These results were corroborated by an independent reprogramming protocol via 4 factor (4F) OSKM reprogramming with individual retroviral plasmids [33] , or through the expression of a Stemcca lentiviral vector encoding 3F OSK (excluding cMyc) ( Supplementary Fig. S2 ). Next, reprogrammed colonies were stained for markers of pluripotency, including Oct4 and Nanog ( Supplementary Fig. S3 ). Nanog staining demonstrates bona fide pluripotency of the iPSC colonies, as it is not encoded by Stemcca. By counting Nanog-positive colonies, we confirmed enhanced reprogramming in the absence of macroH2A isoforms ( Fig. 2f ). Of note, a tandem staining protocol of AP staining followed by Nanog immunofluorescence demonstrated that the majority of AP-positive colonies were fully reprogrammed ( Fig. 2f ). Collectively, these studies suggest that loss of macroH2A isoforms enhances iPS reprogramming. We note here that although macroH2A was reported to be a barrier to Xi reactivation in SCNT studies by Gurdon and colleagues [24] , we show here that macroH2A acts as a barrier to iPS reprogramming independent of its role in X inactivation, as male and female cells reprogram with similar efficiencies ( Fig. 2d–f ). macroH2A2 is the predominant barrier to reprogramming We next inquired which macroH2A variants have a role in the reprogramming process. In order to address this question, we utilized DFs derived from both single (macroH2A1- or macroH2A2-deficient) and dKO mice ( Fig. 3a ). While both single KOs showed a trend toward increased reprogramming, we only observed a significant increase in reprogramming in the dKO DFs ( Fig. 3b ). This suggests that macroH2A1 and macroH2A2 act cooperatively in the reprogramming process. 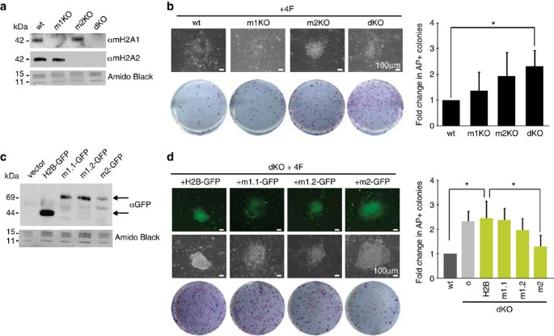Figure 3: macroH2A2 is the predominant epigenetic barrier in reprogramming. (a) Chromatin extracts from wt, macroH2A1 −/− (m1KO), macroH2A2 −/− (m2KO) and dKO DFs probed with macroH2A1 and macroH2A2 antibodies. Amido black of core histones used for loading. (b) Representative wells of AP-positive iPS colonies at 12 days post infection, bright field image of single colonies shown; Scale bar, 100 μm. Quantitation of fold-change in AP-positive colonies over wt (shown right); mean±s.d. (n=4);P-value (asterisk):P=0.002 (wt versus dKO). (c) Chromatin extracts from dKO DFs expressing GFP-tagged macroH2A isoforms (top arrow), H2B-GFP (bottom arrow) and vector alone blotted for GFP. Amido black of core histones used for loading. (d) Representative wells of AP-positive iPS colonies at 12 days post infection, bright field and fluorescence image of individual dKO colonies expressing H2B-GFP and macroH2A GFP-tagged isoforms; Scale bar, 100 μm. Quantitation of fold-change in AP-positive colonies over wt (shown right); [o] represents uninfected; mean±s.d. (n=3); unpaired Student’s test (two tailed)P-value (asterisk):P=0.007 (wt versus dKO+H2B);P=0.036 (dKO+H2B versus dKO+m2). Figure 3: macroH2A2 is the predominant epigenetic barrier in reprogramming. ( a ) Chromatin extracts from wt, macroH2A1 −/− (m1KO), macroH2A2 −/− (m2KO) and dKO DFs probed with macroH2A1 and macroH2A2 antibodies. Amido black of core histones used for loading. ( b ) Representative wells of AP-positive iPS colonies at 12 days post infection, bright field image of single colonies shown; Scale bar, 100 μm. Quantitation of fold-change in AP-positive colonies over wt (shown right); mean±s.d. ( n =4); P -value (asterisk): P =0.002 (wt versus dKO). ( c ) Chromatin extracts from dKO DFs expressing GFP-tagged macroH2A isoforms (top arrow), H2B-GFP (bottom arrow) and vector alone blotted for GFP. Amido black of core histones used for loading. ( d ) Representative wells of AP-positive iPS colonies at 12 days post infection, bright field and fluorescence image of individual dKO colonies expressing H2B-GFP and macroH2A GFP-tagged isoforms; Scale bar, 100 μm. Quantitation of fold-change in AP-positive colonies over wt (shown right); [o] represents uninfected; mean±s.d. ( n =3); unpaired Student’s test (two tailed) P -value (asterisk): P =0.007 (wt versus dKO+H2B); P =0.036 (dKO+H2B versus dKO+m2). Full size image In order to tease apart the role of the macroH2A1 splice variants, macroH2A1.1 and macroH2A1.2, and investigate barrier function by all individual macroH2A isoforms, we ectopically expressed macroH2A1.1, macroH2A1.2 and macroH2A2 as green fluorescent protein (GFP)-fusion proteins in dKO DFs ( Fig. 3c and Supplementary Fig. S4a–c ). Compared with canonical histone H2B, macroH2A2 significantly suppressed the enhanced reprogramming phenotype. While macroH2A1.1 had no effect, macroH2A1.2 showed a slight decrease in reprogramming efficiency ( Fig. 3d ). These data suggest that macroH2A2 acts as the predominant epigenetic barrier, with a potential contribution from macroH2A1.2. Intriguingly, the expression of multiple macroH2A variants simultaneously in dKO DFs (mH2A1.1+mH2A1.2, mH2A1.2+macroH2A2, all three isoforms) did not show significant barrier function, although mH2A1.2+macroH2A2 displayed a slight decrease in AP-positive colonies ( Supplementary Fig. S4d,e ). This might be due to competition between variants or to deregulation of incorporation into chromatin when variants are simultaneously overexpressed. In addition, because only macroH2A1.1 has the ability to bind ADP-ribose [34] , this function may prevent macroH2A1.1 from being involved in creating a barrier for iPS reprogramming and, in turn, inhibit macroH2A1.2 or macroH2A2 function. macroH2A co-localizes genomically with H3K27me3 domains In order to gain insights into the mechanism by which macroH2A isoforms inhibit reprogramming, we hypothesized that their absence might alter the histone post-translational modification (PTM) landscape. By qMS analysis we show that iPS reprogramming affects wt and dKO PTM changes similarly, including a striking increase of H3K27ac and decrease of H3K27me3 levels ( Fig. 4a ; Supplementary Fig. S5 ). H3K27me3 and macroH2A occupancy have similar patterns by ChIP-chip analysis [3] , [5] , and recently, H3K27me3 demethylation (via Utx) was shown to be a key step in iPS reprogramming [35] . Therefore, we further dissected the interplay between macroH2A and H3K27 PTMs. 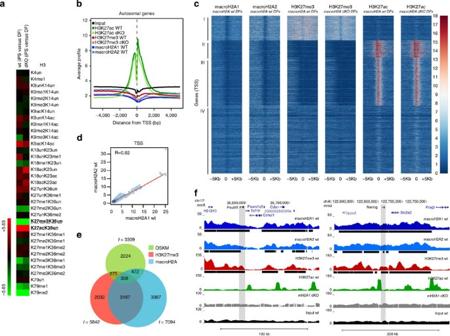Figure 4: macroH2A isoforms and H3K27me3 occupy pluripotency genes in DFs. (a) qMS heatmap with H3 PTMs comparing iPS cells with DFs, in wt and mH2A dKO cells. H3K27me3 and H3K27ac are among the most striking changes upon reprogramming. Two technical replicates run for each of two biological samples. (b) Average signal (100 bp window) of the ChIP-seq read counts normalized to total number of reads (counts per million reads), plotted against the distance (−5 Kb, +5 Kb), from the nearest annotated (USCS mm9) TSS of all autosomal genes. (c) Heatmap of all annotated TSS (−5 Kb, +5 Kb) based on macroH2A1, macroH2A2, H3K27me3 and H3K27ac enrichment in wt and macroH2A dKO DFs, with k-means clustering of all samples (k=4) allowing for four distinct classes of genes (I, II, III, IV). (d) Correlation plot of macroH2A1 and macroH2A2 ChIP-seq reads at the TSS of autosomal genes in wt DFs. Pearson correlation value (R=0.92) indicates a strong correlation between macroH2A1 and macroH2A2. (e) Venn-diagram representing genes enriched in H3K27me3, macroH2A-bound genes (combined macroH2A1 and macroH2A2 targets) and bound by at least one of the four (OSKM) factors37. (f) ChIP-seq profiles (UCSC browser) of two major pluripotency genes (Pou5f1(Oct4)and Nanog)for macroH2A1, macroH2A2, H3K27me3 and H3K27ac; grey bar represents the gene body region. Chromatin domains identified with Sicer annotated under each profile (black bar); macroH2A1 ChIP-seq in dKO DFs and Input used as controls. Figure 4: macroH2A isoforms and H3K27me3 occupy pluripotency genes in DFs. ( a ) qMS heatmap with H3 PTMs comparing iPS cells with DFs, in wt and mH2A dKO cells. H3K27me3 and H3K27ac are among the most striking changes upon reprogramming. Two technical replicates run for each of two biological samples. ( b ) Average signal (100 bp window) of the ChIP-seq read counts normalized to total number of reads (counts per million reads), plotted against the distance (−5 Kb, +5 Kb), from the nearest annotated (USCS mm9) TSS of all autosomal genes. ( c ) Heatmap of all annotated TSS (−5 Kb, +5 Kb) based on macroH2A1, macroH2A2, H3K27me3 and H3K27ac enrichment in wt and macroH2A dKO DFs, with k-means clustering of all samples ( k =4) allowing for four distinct classes of genes (I, II, III, IV). ( d ) Correlation plot of macroH2A1 and macroH2A2 ChIP-seq reads at the TSS of autosomal genes in wt DFs. Pearson correlation value ( R =0.92) indicates a strong correlation between macroH2A1 and macroH2A2. ( e ) Venn-diagram representing genes enriched in H3K27me3, macroH2A-bound genes (combined macroH2A1 and macroH2A2 targets) and bound by at least one of the four (OSKM) factors [37] . ( f ) ChIP-seq profiles (UCSC browser) of two major pluripotency genes ( Pou5f1 (Oct4) and Nanog) for macroH2A1, macroH2A2, H3K27me3 and H3K27ac; grey bar represents the gene body region. Chromatin domains identified with Sicer annotated under each profile (black bar); macroH2A1 ChIP-seq in dKO DFs and Input used as controls. Full size image We next investigated macroH2A1, macroH2A2, H3K27me3 and H3K27ac genomic occupancy by native chromatin immunoprecipitation followed by deep sequencing (ChIP-seq) in wt DFs ( Supplementary Fig. S6 ). We also performed ChIP-seq for K27 PTMs in dKO DFs in order to examine any potential differences in their patterns in the absence of macroH2A (see below; Supplementary Fig. S6 ). Consistent with our previous macroH2A1 ChIP-seq studies in K562 cells, we observed that transcription start sites (TSSs) lack macroH2A isoforms, while macroH2A-containing nucleosomes are present at upstream regulatory regions and/or gene bodies, and that macroH2A1 and macroH2A2 form large domains [10] ( Fig. 4b ; Supplementary Fig. S6b ). We also observed that macroH2A1, macroH2A2 and H3K27me3 followed a similar occupancy pattern around TSSs, while H3K27ac was enriched at TSSs [36] ( Fig. 4b ). Of note, macroH2A1 ChIP in macroH2A dKO cells was performed as a control, generating a very low number of unique alignments and an enrichment pattern similar to Input sample ( Supplementary Fig. S6 ). Based on the ChIP-seq signal around the TSS of the six different data sets (of all annotated autosomal genes), we were able to identify four distinct classes of genes ( Fig. 4c ). Class I in particular, consists of genes bound by macroH2A1 and macroH2A2 that are enriched for H3K27me3, and devoid of H3K27ac ( Fig. 4c and Supplementary Fig. S7a ; see below). In this class of genes, there is strong macroH2A enrichment both upstream and downstream of the TSS, which we have previously shown to associate with transcriptionally repressed genes [10] . Next, by comparing all ChIP-seq reads using a pair-wise correlation analysis, we observed a striking correlation between macroH2A1 and macroH2A2 (Pearson correlation R =0.92 for TSS; R =0.94 for genome-wide) ( Fig. 4d and Supplementary Fig. S7b ). We therefore combined macroH2A1 and macroH2A2 target genes (referred to as macroH2A-bound genes), for further analysis. Hierarchical clustering also confirmed a correlation between both macroH2A isoforms and H3K27me3, while none of these repressive marks positively correlate with H3K27ac ( Supplementary Fig. S7b ). Interestingly, we did not observe a significant difference in enrichment of H3K27me3 and H3K27ac in the absence of macroH2A, as calculated using a Pearson correlation for the samples in wt and macroH2A dKO DFs ( Fig. 4c , Supplementary Fig. S7c ). Collectively, global analysis of our ChIP-seq data demonstrates the following: (i) a striking genome-wide correlation between macroH2A1 and macroH2A2, which correlates with H3K27me3 and (ii) the absence of macroH2A isoforms does not globally alter H3K27 PTMs in the ground state of DFs. macroH2A occupies genes encoding pluripotency regulators In order to probe the role of macroH2A as a barrier to reprogramming, we queried its presence at genes bound by at least one of the 4F (OSKM) [37] . These factors activate the ESC-specific transcriptional network through their binding mostly at promoter regions [37] . We found that macroH2A is present at ~24% (810/3309) of OSKM-bound genes, while H3K27me3 occupies ~18% (613/3309) in DFs ( Fig. 4e ). Next, we investigated the profiles of the master regulators of pluripotency. By examining the Oct4 (Pou5f1) and Nanog loci, using the UCSC browser, a macroH2A/H3K27me3 domain is evident ( Fig. 4f ). Such domains often span large regions of up to 100–200 kb, encompassing multiple genes and their regulatory regions. Next, we confirmed the macroH2A landscape at the Pou5f1 locus (which encodes Oct4 ) by ChIP-quantitative PCR (qPCR) analysis. We observed a peak of macroH2A1 enrichment upstream of the transcriptional start site (TSS) at the enhancer elements of Pou5f1 ( Supplementary Fig. S8a ). The distal enhancer (−2 Kb) is a site where the pluripotency TFs bind and regulate Oct4 expression in ESCs [38] . ChIP analysis of Oct4 itself, Nanog and Sox2 demonstrates distinct binding at the −2 kb position in ESCs ( Supplementary Fig. S8b ). Furthermore, we performed ChIP analysis for macroH2A1 at the distal enhancer element in ESCs undergoing differentiation, which shows macroH2A1 deposition upon RA differentiation ( Supplementary Fig. S8c ), and is consistent with its global chromatin deposition ( Fig. 1 ). macroH2A is enriched at Utx target genes The studies above suggested that macroH2A and H3K27me3 might work together in reinforcing silent states of pluripotency genes in differentiated cells. These data, combined with an SSEA1-positive population early in the reprogramming process in macroH2A dKO cells ( Fig. 2d ), led us to query published data sets describing genes induced early in reprogramming. Recently the H3K27me3 histone demethlyase, Utx, was described as a critical enzyme in the induction of iPS reprogramming [35] . Utx regulates the reactivation of a class of ~1400 genes that are transcriptionally upregulated in the early stages of reprogramming. Of these genes a subset of ~100 genes had aberrantly high levels of H3K27me3 in Utx -depleted cells, suggesting their reactivation was inhibited by retention of H3K27me3. By overlaying our ChIP-seq data onto Utx targets with aberrant H3K27me3 [35] , we found that Utx targets are composed primarily of Class I genes, which are enriched for macroH2A and H3K27me3 ( Fig. 5a ). Next, we compared macroH2A, H3K27me3 and H3K27ac ChIP-seq data sets with the gene sets that displayed either normal or aberrant H3K27me3 levels. In keeping with the findings of Hanna and colleagues [35] , we find marked enrichment of H3K27me3 (88%) at the aberrantly methylated genes in wt DFs ( Fig. 5b ). Our analysis also revealed a striking enrichment of macroH2A-bound genes at these Utx target genes (75%), which contains TFs such as Sall1 and Sall4 ( Fig. 5b ). Using the UCSC browser, we observed distinct macroH2A/H3K27me3 domains at these pluripotency promoting factors ( Fig. 5c ). 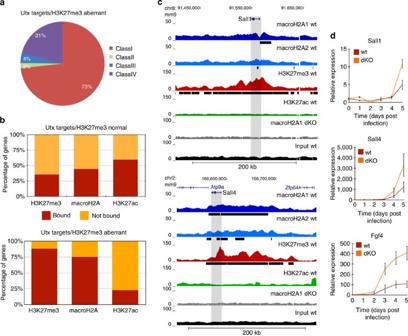Figure 5: macroH2A occupancy inhibits activation of Utx target genes required early in iPS reprogramming. (a) Pie chart of Utx target genes with aberrant H3K27me3 methylation (inUtxKO)35composed of the four classes of genes fromFig. 4c. (b) Comparison of genes marked by H3K27me3, H3K27ac and macroH2A-bound genes (combined macroH2A1 and macroH2A2 targets) in wt DFs and genes reactivated early in iPS reprogramming with normal H3K27me3 demethylation inUtxKO cells (top) versus genes that aberrantly retain H3K27me3 inUtxKO cells (bottom)35. MacroH2A is enriched in genes that are unable to demethylate H3K27me3 in the absence ofUtx. (c) ChIP-seq profile (UCSC browser) of two genes bound by macroH2A1, macroH2A2 and H3K27me3 in DFs that are not properly demethylated in the absence ofUtxduring reprogramming (Sall1 and Sall4-grey bar represents the gene body region). Chromatin domains identified with Sicer annotated under each profile (black bar). MacroH2A1 ChIP-seq in dKO DFs and Input used as controls. (d) Time course analysis of mRNA expression of three Utx target genes (Fgf4, Sall1 and Sall4) during reprogramming shows delayed induction in wt DFs as compared with macroH2A dKO DFs. Relative expression is plotted using ribosomal L7 as a house-keeping gene, and compared with DFs at day 0, mean±s.d. (n=3). Figure 5: macroH2A occupancy inhibits activation of Utx target genes required early in iPS reprogramming. ( a ) Pie chart of Utx target genes with aberrant H3K27me3 methylation (in Utx KO) [35] composed of the four classes of genes from Fig. 4c . ( b ) Comparison of genes marked by H3K27me3, H3K27ac and macroH2A-bound genes (combined macroH2A1 and macroH2A2 targets) in wt DFs and genes reactivated early in iPS reprogramming with normal H3K27me3 demethylation in Utx KO cells (top) versus genes that aberrantly retain H3K27me3 in Utx KO cells (bottom) [35] . MacroH2A is enriched in genes that are unable to demethylate H3K27me3 in the absence of Utx . ( c ) ChIP-seq profile (UCSC browser) of two genes bound by macroH2A1, macroH2A2 and H3K27me3 in DFs that are not properly demethylated in the absence of Utx during reprogramming (Sall1 and Sall4-grey bar represents the gene body region). Chromatin domains identified with Sicer annotated under each profile (black bar). MacroH2A1 ChIP-seq in dKO DFs and Input used as controls. ( d ) Time course analysis of mRNA expression of three Utx target genes (Fgf4, Sall1 and Sall4) during reprogramming shows delayed induction in wt DFs as compared with macroH2A dKO DFs. Relative expression is plotted using ribosomal L7 as a house-keeping gene, and compared with DFs at day 0, mean±s.d. ( n =3). Full size image To address the role of macroH2A occupancy at these genes, we probed the kinetics of pluripotency gene activation during reprogramming. Using quantitative reverse transcription–PCR (qRT–PCR) analysis, we compared the activation of multiple Utx target genes that are also bound by macroH2A in both wt and mH2A dKO DFs. Indeed, the absence of macroH2A leads to a more robust, and in some cases, an earlier transcriptional activation of such genes ( Fig. 5d ). Collectively, our data suggests that macroH2A and H3K27me3 cooperate in repressing pluripotency factors in differentiated cells and must be removed upon reprogramming to reactivate a critical set of early iPS-induced genes. Absence of macroH2A does not impair pluripotency Next, we queried whether macroH2A isoforms have a significant role in differentiation. Therefore, as depicted in Fig. 2c , iPSC colonies were picked and expanded in order to generate both wt and dKO iPSC lines. These cells were treated with a Cre recombinase-expressing adenovirus to remove the Stemcca cassette ( Supplementary Fig. S9a ). Using these lines, we investigated pluripotency potential in the absence of macroH2A isoforms. Both wt and dKO iPSCs grew similarly to ESCs, without signs of spontaneous differentiation ( Fig. 6a ; bright field). In addition, AP and Nanog-positive staining was observed in both dKO and wt iPSCs ( Supplementary Fig. S9b ). Next, we examined the reactivation of the Xi, a hallmark of fully reprogrammed iPSCs [39] , through H3K27me3 staining. Neither the wt nor the dKO iPSCs (two female lines of each examined) showed evidence of an Xi ( Supplementary Fig. S9b ). Therefore, the dKO cells displayed ESC-like features such as self-renewal, expression of pluripotency markers, and showed no evidence of Xi chromosomes. These results are consistent with recently published studies whereby loss of macroH2A isoforms in ESCs (via shRNAs) did not show evidence of a compromised ESC state [18] , [19] . 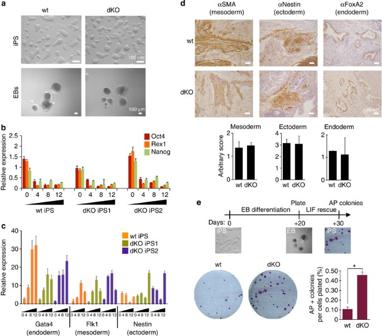Figure 6: macroH2A dKO iPS cells are pluripotent and retain stem-like plasticity. (a) Bright field of iPS cells and EBs (day 12) derived from wt and dKO DFs display no morphological differences; Scale bar, 100 μm. (b) Expression of pluripotency regulators (Oct4, Rex1 and Nanog) was analysed by qPCR during EB differentiation for the course of 12 days; relative expression is plotted using ribosomal L7 as a house-keeping gene, and compared with ESC levels, mean±s.d. (n=3). (c) Expression of differentiation markers was analysed by qPCR during EB differentiation showing upregulation of lineage markers of all three germ layers. Relative expression is plotted using ribosomal L7 as a house-keeping gene, and compared with ESC levels, mean±s.d. (n=3). (d) IHC of representative wt and dKO teratomas derived from iPSCs, probing for mesoderm (SMA), ectoderm (Nestin) and endoderm (FoxA2). Each cross section was scored by number of positively stained structures per slide, mean±s.d. (n=3) Scale bar, 100 μm. No statistical differences were observed upon quantification of staining (below). (e) Experimental scheme of LIF rescue analysis shown on top. Numbers of AP-positive colonies were analysed after 7–10 days. Quantification of AP-positive colonies per number of cells plated, mean±s.d. (n=3); unpaired Student’s test (two tailed)P=0.0002 (asterisk); representative wells shown. Figure 6: macroH2A dKO iPS cells are pluripotent and retain stem-like plasticity. ( a ) Bright field of iPS cells and EBs (day 12) derived from wt and dKO DFs display no morphological differences; Scale bar, 100 μm. ( b ) Expression of pluripotency regulators (Oct4, Rex1 and Nanog) was analysed by qPCR during EB differentiation for the course of 12 days; relative expression is plotted using ribosomal L7 as a house-keeping gene, and compared with ESC levels, mean±s.d. ( n =3). ( c ) Expression of differentiation markers was analysed by qPCR during EB differentiation showing upregulation of lineage markers of all three germ layers. Relative expression is plotted using ribosomal L7 as a house-keeping gene, and compared with ESC levels, mean±s.d. ( n =3). ( d ) IHC of representative wt and dKO teratomas derived from iPSCs, probing for mesoderm (SMA), ectoderm (Nestin) and endoderm (FoxA2). Each cross section was scored by number of positively stained structures per slide, mean±s.d. ( n =3) Scale bar, 100 μm. No statistical differences were observed upon quantification of staining (below). ( e ) Experimental scheme of LIF rescue analysis shown on top. Numbers of AP-positive colonies were analysed after 7–10 days. Quantification of AP-positive colonies per number of cells plated, mean±s.d. ( n =3); unpaired Student’s test (two tailed) P =0.0002 (asterisk); representative wells shown. Full size image Next, the pluripotency of wt and macroH2A dKO iPSCs was challenged. Differentiation was induced via EB formation assays, and similar morphology was observed between the two genotypes ( Fig. 6a ). To further examine the EB differentiation, we dissected the gene expression profiles of both pluripotency genes and lineage markers of all three germ layers. qRT–PCR demonstrated a drop in expression of pluripotency markers Nanog, Oct4 and Rex1 with similar kinetics in both wt and dKO cells (as to ESCs), suggesting that loss of macroH2A does not affect silencing of these genes ( Fig. 6b ). Although macroH2A is deposited at pluripotency genes (such as Pou5f1 ) during differentiation ( Supplementary Fig. S8c ), they are also silenced by additional mechanisms such as H3K27me3, as well as H3K9me3 and DNA methylation [40] , [41] . This suggests that macroH2A is not required for initial silencing of pluripotency genes, but may act to maintain silencing in coordination with other silencing mechanisms, akin to its role at the Xi [4] . We also examined the kinetics of lineage marker expression towards the three germ layers upon EB differentiation. This analysis displayed remarkable similarity between wt and dKO iPSCs ( Fig. 6c ). We surveyed the expression of at least three markers of each lineage, endoderm, mesoderm and ectoderm ( Fig. 6c , Supplementary Fig. S10a–c ). Moreover, wt iPSCs show deposition of macroH2A1 and macroH2A2 in the chromatin fraction upon differentiation, with similar kinetics to ESCs ( Fig. 1c ), while macroH2A dKO cells display no signals, as expected ( Supplementary Fig. S10d ). Chromatin-bound levels of both Oct4 and H2A.Z decreased in a similar fashion in wt, dKO cells, and ESCs ( Supplementary Fig. S10d ; Fig. 1c ). Next, wt and dKO iPSCs were injected into immunodeficient mice for teratoma analysis. Here we observed formation of all three germ layers from both wt and dKO cells by hematoxylin and eosin staining ( Supplementary Fig. S10e ). Using antibodies specific for mesodermal (Smooth-Muscle Actin), neuroectodermal (Nestin) and endodermal (FoxA2) lineages, we performed immunohistochemistry (IHC) and quantified positively stained structures in both wt and macroH2A dKO iPS-derived teratomas ( Fig. 6d ). No significant differences were observed between wt and macroH2A dKO cells for any of the lineage markers ( Fig. 6d ). Collectively, our pluripotency studies indicate that the absence of macroH2A isoforms does not compromise the self-renewal or differentiation potential of dKO iPSCs. To assess the capacity of such differentiated cells to return back to an ESC-like state, differentiated EBs (day 20) were then challenged in ESC media in the presence of leukemia inhibitory factor (LIF). After one week, the number of colonies formed per cell plated was determined ( Fig. 6e ). Consistent with our iPS reprogramming studies, we find that EB differentiated cells lacking macroH2A showed an increased ability to form AP-positive colonies, even after a prolonged period of differentiation, suggesting they retain stem-like plasticity. In recent years, there has been an overwhelming interest in pluripotent ESCs because of their potential to understand developmental processes and treat human disease [42] . Therefore, the ability to reprogram somatic cells to a pluripotent state, particularly by iPSC methodologies, has generated much excitement [43] . Yet despite its potential impact, the molecular mechanisms of reprogramming, especially as they relate to chromatin biology, remain unclear. Recent studies have begun to address the role of chromatin factors during reprogramming, such as Chd1 [44] ,the BAF [45] complex and Wdr5 [46] . Interestingly, many of the global PTM changes that we found by our qMS analysis of iPSCs versus DFs ( Fig. 4a ), have recently been described to be necessary for iPS reprogramming. These include loss of K79me2/3 (via antagonizing Dot1L methyltransferase) [47] , loss of K36me2/3 (mediated by Kdm2b) [48] , loss of H3K9me2/3 (via antagonizing Suv39H1 or G9a methyltransferases) [47] , [49] and relevant to this study, loss of H3K27me3 (mediated by Utx) [35] . Moreover, increased global levels of acetylation such as H3K27ac and H3K9ac were also detected by qMS, and are modulated through inhibition of HDACs [27] ( Fig. 4a ; Supplementary Fig. S5 ). However, little is known of the role of histone variants in the context of iPS reprogramming. Here we demonstrate that macroH2A acts as a barrier to iPSC reprogramming. Our findings are consistent with the role of macroH2A in SCNT, albeit with differences depending on the recipient species [22] , [24] . First, macroH2A is rapidly removed from the mammalian somatic cell nucleus upon transplantation into mouse oocytes, suggesting that its presence creates a barrier to genome-wide reprogramming [22] . In the Xenopus model system, macroH2A presence correlates with a lack of Xi reactivation, suggesting it acts as a barrier at this specialized domain of heterochromatin [24] . Finally, Pasque et al [50] . recently demonstrated an inhibitory role for macroH2A isoforms in iPS reprogramming using RNA interference approaches. Here we have explored the genomic landscape of macroH2A and demonstrated that macroH2A1 and macroH2A2, along with H3K27me3, are physically present at pluripotency genes in differentiated cells. Notably, macroH2A deposition is significantly enriched at Utx target genes, which are critical during the early stages of reprogramming. In fact, in macroH2A dKO cells, the expression of SSEA1 (an early marker of reprogramming) was significantly increased when compared with wt fibroblasts ( Fig. 2d ). This suggests that loss of macroH2A isoforms facilitates the early stages of reprogramming upon ectopic OSKM (and OSK) expression, possibly by allowing for more efficient chromatin remodelling or facilitating demethylation of H3K27me3. Consistent with this, our kinetic studies during reprogramming suggest that Utx target genes are more efficiently reactivated in macroH2A dKO DFs than in wt cells ( Fig. 5d ). Despite the strong correlation between macroH2A-bound genes and H3K27me3, the absence of macroH2A isoforms does not affect H3K27me3 localization in DFs, suggesting a redundancy between the two repressive modifications. Although the mechanism by which macroH2A gets deposited in chromatin is unknown (ATRX negatively regulates macroH2A deposition [10] ), its chromatin incorporation may be important to stabilize H3K27me3 at pluripotency genes during reprograming, thus acting as a barrier. Alternatively, since aberrantly methylated Utx target genes are also bound by macroH2A1 and macroH2A2, it is possible that H3K27me3-containing nucleosomes are a flag for macroH2A deposition. Here we propose that macroH2A isoforms provide a redundant silencing layer at pluripotency genes that, in turn, presents as an epigenetic barrier when differentiated cells are challenged to reprogram ( Fig. 7 ). Our data shows that macroH2A is not required for the initial silencing of pluripotency genes during differentiation, but is incorporated into pluripotency gene regulatory sites during the process. This is similar to the late deposition of macroH2A at the Xi, and suggests that formation of a multi-layered barrier prevents reactivation of unwanted genes in a somatic cell that might trigger alternative cell fates. In turn, we find that while cells derived from the genetically deficient macroH2A mouse model display enhanced reprogramming, they do not showed impaired differentiation. This is in contrast with a recent study where depletion of macroH2A isoforms in ESCs via RNA interference showed differentiation defects [18] . These differences may be attributed to the approaches used (knockout versus knockdown) or technicalities of the differentiation methods used. 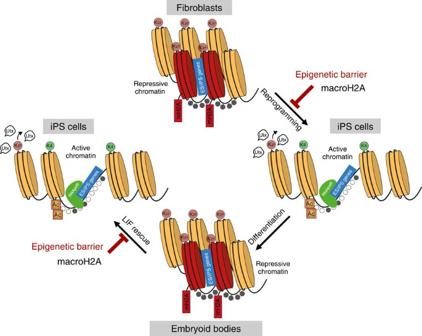Figure 7: The histone variant macroH2A acts as a barrier to somatic cell reprogramming. macroH2A is enriched in somatic cells enabling pluripotency genes to be maintained in a repressed state in differentiated cells. This deposition is correlated with enrichment of the repressive mark H3K27me3. Upon overexpression of reprogramming factors in differentiated cells, macroH2A provides an extra layer of silencing at pluripotency genes, and therefore acts as a barrier to reprogramming. The histone demethylase Utx is required to remove H3K27me3 at a subset of genes, also bound by macroH2A, that need to be reactivated upon reprogramming. Differentiation of pluripotent stem cells is not impaired in the absence of macroH2A, as it likely acts as a final ‘lock’ upon other silencing mechanisms. However, differentiated cells (for example, EBs) lacking macroH2A are more amenable to reactivation of the pluripotent state, further suggesting that its presence induces a barrier to reprogramming in differentiated cells. Figure 7: The histone variant macroH2A acts as a barrier to somatic cell reprogramming. macroH2A is enriched in somatic cells enabling pluripotency genes to be maintained in a repressed state in differentiated cells. This deposition is correlated with enrichment of the repressive mark H3K27me3. Upon overexpression of reprogramming factors in differentiated cells, macroH2A provides an extra layer of silencing at pluripotency genes, and therefore acts as a barrier to reprogramming. The histone demethylase Utx is required to remove H3K27me3 at a subset of genes, also bound by macroH2A, that need to be reactivated upon reprogramming. Differentiation of pluripotent stem cells is not impaired in the absence of macroH2A, as it likely acts as a final ‘lock’ upon other silencing mechanisms. However, differentiated cells (for example, EBs) lacking macroH2A are more amenable to reactivation of the pluripotent state, further suggesting that its presence induces a barrier to reprogramming in differentiated cells. Full size image In closing, deciphering the regulation of transcriptional programs during development by incorporation of histone variants may broaden our perspectives on cell identity, that is, by restricting cellular plasticity in the case of macroH2A, or by modulating cellular memory, as has been suggested for the H3 variant H3.3 (ref. 51 ). As macroH2A has been implicated as a tumour suppressor [52] , [53] , these new avenues may also enhance our understanding of cancer biology. Cell culture DFs, MEFs, and HEK293 cells were grown in DMEM (CellGro) with 10% FBS and 1% Penicillin/Streptomycin CCE ESCs (ES cell line derived from a male 129/Sv mouse strain), E14 (ES cell line derived from a male 129/Ola mouse strain) and iPSCs were maintained in standard ES media (see Supplementary Materials and Methods for details). Plasmids The 4F (Oct4, Sox2, Klf4 and Myc) used for iPS reprogramming are encoded in a polycystronic lentiviral vector (Stemcca, kindly provided by Gustavo Mostoslavsky, Boston University). Human H2B-GFP is encoded in pLKO.1, and GFP-tagged rat macroH2A1.1, rat macroH2A1.2 and human macroH2A2 constructs were cloned into this same plasmid. Differentiation procedures For RA differentiation, ESCs were plated on 0.1% gelatin coated plates at a density of 5 × 10 4 . The next day, LIF was removed and 2 μM of RA was administered. EBs were formed by plating 1 × 10 6 cells into low attachment conditions (suspension culture) in ES media without LIF. DF isolation Pregnant females of known genotype were individually caged on day E18.5. Pups were killed following the Institutional Animal Care and Use Committee (IACUC) guidelines (protocol # 803525, University of Pennsylvania), and skins were carefully removed and placed in sterile PBS. Pups were sexed by checking the presence of the male or female gonads and were grouped according to their sex. Skins were placed with the dermal side down into a sterile 35 mm petri dish and floated in 0.25% trypsin-EDTA overnight in 4 °C. The following day, the epidermis was removed and dermis was incubated in 0.2% collagenase in DMEM for 1 h at 37 °C. The dermis was shaken to release the fibroblasts, and this mixed cell population was pelleted and plated in DMEM with 10% FBS, 1% P/S, 2.5 units ml −1 Amphotericin B, and 2 mM L -Glutamine. Calcium was raised to 6 mM to induce calcium-dependent differentiation and detachment of contaminating keratinocytes. iPS reprogramming iPS reprogramming was performed as described [33] with slight modifications. Early passage DFs were plated on DMEM with 10% FBS and 1% Penicillin/Streptomycin 1 day before infection according to the well surface area (10 000 cells on a 24-well plate, 50 000 cells on a 6-well plate or 500 000 on a 100-mm dish). Cells were infected by adding ultra-concentrated virus, with fresh media and 8 ng μl −1 Polybrene (Millipore) overnight. For overexpression of the GFP-tagged histones, cells were plated as described above, and infected the following day. Two days later they were passaged and infected with 4F the following day. ESC media was added 2 days after infection, and 4–5 days post infection the cells were trypsinized and re-plated onto 6-well plates with inactivated MEFs. AP staining was performed according to the manufacturer’s protocol (Stemgent). Immunofluorescence for Nanog was performed on 6-well plates after AP staining, as described below. SSEA1 staining was performed using a mouse monoclonal anti-SSEA-1 antibody conjugated to Phycoerythrin, and was performed according to the manufacture’s protocol (R&D). Staining was analysed by FACS on a LSRII machine and data was analysed with Flowjo. Chromatin fractionation and histone acid extraction Procedures performed as described [10] . Quantitative Mass Spectrometry qMS was performed as described [53] , [54] . Immunofluorescence and immunoblots Immunoblots were performed as described [10] . For immunofluorescence, ESCs, iPSCs or DFs were plated on chamber glass slides precoated with Matrigel (BD Biosciences). Immunofluorescence was performed as described [44] . Fluorescently conjugated secondary antibodies were subsequently used Alexa-488/594 (Molecular Probes). Nuclei were counterstained with 4',6-diamidino-2-phenylindole (DAPI) and slides were mounted in vectashield (Vector Laboratories). Images presented were acquired on a Zeiss Imager Z1 microscope via deconvolution of 20–30 Z-stack projections using the AxioVision 40 Version 4.8.1.0 software, or were taken from a single projection. For a full list of antibodies used, please see Supplementary Materials and Methods. complementary DNA isolation and qPCR RNA was extracted with the QIAGEN RNeasy Mini Kit. A total of 1 μg of RNA was used to synthesize complementary DNA (cDNA) using Superscript II and Oligo d(T) primers (Invitrogen). qPCR and mRNA analysis was carried out as described [44] . cDNA expression was normalized to L7 levels. Primer sequences are provided in Supplementary Materials and Methods. Native Chromatin Immunoprecipitation and ChIP-seq Native mH2A1 ChIP (Abcam, ab37264), H3K27me3 (Millipore, 07-449) and H3K27ac (Abcam 4729) was performed in wt and macroH2A dKO male DFs; macroH2A2 (Bernstein lab) was performed in wt and dKO female DFs. Input DNA was also prepared and subsequent sequencing on all samples was performed using Illumina Hi-Seq as described [10] . qPCR on ChIP DNA was performed as described above. Primer sequences are provided in Supplementary Materials and Methods. ChIP-seq data analysis Sequence reads were aligned to the mouse genome NCBI build 37 (UCSC, mm9) using Bowtie short read aligner [55] (v 0.12.7), with the following parameters: seed of 50 bp, maximum two mismatches, suppression ( m )=20, and reported alignments ( k )=20. Wiggle files (HAFEZ, unpublished pipeline D.H.), were generated using a 500-bp window sliding 250 bp, counting the number of aligned reads (5′-end of each aligned read), for both ChIP and Input samples. The number of alignments from each window was normalized to the total number of alignments and scaled by factor of 10 7 , to allow comparison between different samples. MACS software [56] (v 1.4.1) was used to identify peaks ( P -value cutoff=1.00e-04 (5e-5 for K27me3 and K27Ac; 5e-3 for mH2A1; 5e-4 for mH2A2), (bw)=300). Genes bound by either macroH2A1, macroH2A2, H3K27me3 or H3K27ac were found by Peak2Gene [57] software tool ( www.cistrome.org ), allowing a span of 5 kb upstream or downstream of the peak. Analysis of histone variants/chromatin modifications with enrichment in broad domains was performed using Sicer [58] (Window 200 bp, Gap 200 bp, fragment size 150 bp, P -value cutoff=0.01). TSS analysis The relative positions of aligned reads to the TSS were generated using RefSeq gene annotations downloaded from the UCSC genome browser (mm9). Analysis of reads distribution around the TSS (+5 Kb and −5 Kb) was performed with a sliding window (100 bp) using the SitePro tool from Cistrome [57] ( www.cistrome.org ). Correlation analysis of ChIP-seq data Hierarchical clustering and correlation coefficient values between samples (genome scale or around the TSS) was performed using the integrative analysis tool from Cistrome [57] ( www.cistrome.org ), with a size window of 100 Kb. Heatmap of the enrichment of each sample in all annotated TSSs (+5 Kb and −5 Kb) was generated using Heatmap from Cistrome [57] ( http://www.cistrome.org) with k-means clustering of four classes calculated amongs all samples. TSS analysis of the four classes of genes was performed using the SitePro tool from Cistrome [57] ( http://www.cistrome.org ) with 100 bp resolution. Venn Diagrams and other comparative analysis were performed with an R script using macroH2A-bound genes (combined macroH2A1 and macroH2A2 targets) and the genes enriched in H3K27me3 and H3K27ac (our data sets), and previously published data on genes bound by OSKM [37] , and early reprogramming/Utx target genes [35] . Data deposition All ChIP-Seq data sets deposited to NCBI’s Gene Expression Omnibus with the deposition number GSE40813. Cross-linked ChIP-qPCR Formaldehyde fixed ChIP was carried out essentially as described [53] with the following antibodies: macroH2A1 (Abcam, ab37264), Nanog (Cosmo Bio, REC-RCAB0002P-F), Oct4 (Santa Cruz, sc8628), Sox2 (Santa Cruz, sc17320) and IgG (Millipore, 12–370). Teratoma Formation Three different dilutions of iPSCs were used to inject subcutaneously into NOD/SCID mice (0.1 × 10 6 , 0.5 × 10 6 , 1 × 10 6 ) using a 1:1 solution of DMEM and Matrigel (BD Biosciences). After 6–8 weeks, teratomas were harvested and fixed in 10% formalin overnight. Samples were then embedded in paraffin, and sections were stained with hematoxylin and eosin (Histopathology Core, Mount Sinai School of Medicine).IHC was performed using antibodies against alpha-SMA (mesoderm) and FoxA2 (endoderm) as described [53] . Nestin staining (ectoderm) was performed using MOM kit (Vector labs). IHC images (10 per antibody stain, per section) were taken on a Nikon E-600 microscope with NIS Elements software (Nikon). Images were scanned and quantified for the number of individual structures/clusters of cells positive by HRP-staining. Three tumours were analysed per condition. LIF rescue assay Differentiated EBs (day 20) were washed with PBS, trypsinized, and resuspended in ESC media. Cells were plated at 5,000, 10,000 or 15,000 cells per gelatinized plate. After 7–10 days, colonies were fixed and stained for AP (Stemgent). The number of colonies were counted and plotted as percentage of AP-positive colonies per cells plated. How to cite this article: Gaspar-Maia, A. et al . MacroH2A histone variants act as a barrier upon reprogramming towards pluripotency. Nat. Commun. 4:1565 doi: 10.1038/ncomms2582 (2013).